Siberian larch forests and the ion content of thaw lakes form a geochemically functional entity Siberian larch forests growing on shallow permafrost soils have not, until now, been considered to be controlling the abiotic and biotic characteristics of the vast number of thaw-lake ecosystems. Here we show, using four independent data sets (a modern data set from 201 lakes from the tundra to taiga, and three lake-core records), that lake-water geochemistry in Yakutia is highly correlated with vegetation. Alkalinity increases with catchment forest density. We postulate that in this arid area, higher evapotranspiration in larch forests compared with that in the tundra vegetation leads to local salt accumulation in soils. Solutes are transported to nearby thaw lakes during rain events and snow melt, but are not fully transported into rivers, because there is no continuous groundwater flow within permafrost soils. This implies that potentially large shifts in the chemical characteristics of aquatic ecosystems to known warming are absent because of the slow response of catchment forests to climate change. In studies on the ecological impacts of global warming, research has concentrated on the role of thaw lakes in the regional organic carbon cycle as sedimentary sinks [1] and as methane sources [2] . Their role in salt and inorganic carbon cycling within the permafrost ecosystems has not, however, been investigated. Larch forests, the major vegetation cover of Siberia ( Fig. 1 ), are assumed to protect permafrost soils from thawing. Permafrost in turn creates a high water table that allows larch forests to grow, even under strongly arid conditions [3] . It has been ignored that such a coupled system can cause strong epigenetic salt accumulation because of the following mechanisms. First, precipitation, representing the major ion source in central Yakutia, continuously contributes dissolved ion input of about 8–19 mg l −1 (mainly SO 4 2− , HCO 3 − , Na + , Ca 2+ and Mg 2+ ) [4] . In addition, some ions are delivered from the soil weathering, although the rate is low [5] . Second, potential evapotranspiration exceeds precipitation. This particularly applies to the central Yakutian lowlands where there is a two-fold higher potential evaporation relative to the actual precipitation [6] . Third, no continuous groundwater flow exists that connects the remote forest sites with the river systems and, thus, the minerals are not permanently removed from the forest sites. As a result, frozen pale soils with a diagnostic illuvial carbonate and salt horizon have developed, particularly in the lowlands [6] . However, despite aridity, the soluble salt content is rather low (also indicated by the growth of Larix , which tolerates only moderate salt levels [7] ). These characteristics inhibit the feedback-driven functional chain from salt accumulation, through forest retreat and enhanced soil warming, to permafrost decay. Hence, the question arises what are the mechanisms that result in low salt and carbonate contents in Larix forests. 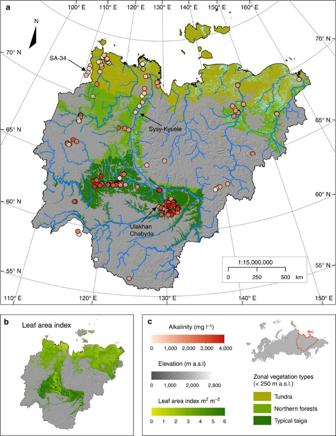Figure 1: Study area in Yakutia. (a) The distribution of zonal vegetation types in the lowlands (<250 m a.s.l.) of Yakutia; also indicated are the 201 sampling sites and measured alkalinity (HCO3−mg l−1). Sites of sediment core studies are indicated by arrows. (b) Satellite-derived leaf-area index of the vegetation period (mean 10 July 2000–10 August 2009) of the Yakutian lowlands34. (c) The outline of Yakutia and its location in Eurasia. Figure 1: Study area in Yakutia. ( a ) The distribution of zonal vegetation types in the lowlands (<250 m a.s.l.) of Yakutia; also indicated are the 201 sampling sites and measured alkalinity (HCO 3 − mg l −1 ). Sites of sediment core studies are indicated by arrows. ( b ) Satellite-derived leaf-area index of the vegetation period (mean 10 July 2000–10 August 2009) of the Yakutian lowlands [34] . ( c ) The outline of Yakutia and its location in Eurasia. Full size image Using four independent data sets, we show that Larix forests, permafrost and the degree of ion content of thaw lakes form an interdependent entity ( Fig. 2 ), which can be described by the following conceptual model. Larix growth in summer is largely limited by the soil moisture [8] . However, interannual variations in evapotranspiration in Larix forests are low, as the trees use meltwater from lower soil depths (supplied as rain during the previous summer) [3] , [9] . To avoid overconcentration in tissues during water uptake, plants actively leave ions in the rooting zone [10] . Salts are temporally stored in the soil and solutes are washed into thermokarst depressions (alases) with spring meltwater [11] or during wet summers [3] , [9] . Accordingly, Larix forest soils show a much lower salt content than grassland soils in the alases, despite a higher evapotranspiration in forests [9] , [12] . This implies that epigenetic accumulated salt in permafrost depressions does not only originate locally but is also continuously supplied from the surrounding forests. The strength of long-term salt accumulation in thaw lakes is, together with the frequency of lake drainage or (where occurring) outflow volume, a function of the strength of evapotranspiration in addition to evaporation from the lake surface. The strength of evapotranspiration (which is related to the relative contribution of latent heat in the energy budget) is primarily a function of the photosynthetically active leaf area ( Fig. 1 ) and, therefore, increases markedly across the tundra–taiga ecotone [13] , as confirmed by the land-surface model results for Yakutia [14] . 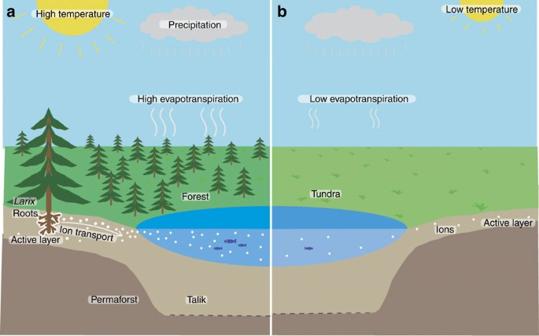Figure 2: Conceptual model visualization. We assume that in the forest sites (panela) due to higher evapotranspiration, relative to tundra sites (panelb), and a lag in a continuous groundwater flow due to permafrost, ions supplied by precipitation become enriched in nearby thermokarst lakes. Figure 2: Conceptual model visualization. We assume that in the forest sites (panel a ) due to higher evapotranspiration, relative to tundra sites (panel b ), and a lag in a continuous groundwater flow due to permafrost, ions supplied by precipitation become enriched in nearby thermokarst lakes. Full size image Modern lake chemistry and forest–tundra transition in space The Yakutian lowlands, where ice-rich permafrost produces strong thermokarst processes [15] , have one of the highest thaw-lake densities. According to our 201 lake data set ( Fig. 1 ), most lakes are shallow but the total ion content and alkalinity are highly variable ( Table 1 ). According to our conceptual model, the tundra–forest transition in space today should be paralleled by an increase in ion content in thaw lakes. We find that the present-day lake water chemistry is significantly related to the remote sensing-derived leaf-area index in lake catchments, that is, the leaf-area index uniquely explains more variation in water ion composition than July temperature or lake morphological parameters do in redundancy analyses (RDA, Table 2 , Supplementary Fig. S1 ), the multivariate analogue to multiple linear regression (see Methods). RDA reveals that of the 13.0% of the total explained variation in the modern diatom spectra from these lakes ( Table 2 ); 10.5% is uniquely explained by a representative set of chemical variables (HCO 3 − , Cl − and Si), whereas the morphological variables explain a much lower percentage (2.4%). Among the chemical variables, alkalinity explains the most variation, indicating its potential for palaeoecological reconstructions ( Supplementary Figs S2 and S3 , and Supplementary Table S1 ). Table 1 Characteristics of sampled lakes and vegetation type for the Yakutian lowlands. Full size table Table 2 Results of redundancy analyses. Full size table Lake Sysy Kyuele core and Holocene forest–tundra transition We have investigated the Holocene vegetation and alkalinity changes from a sediment core from the Lake Sysy Kyuele ( Figs 1 and 3a ) located in the northern Lena River lowlands presently surrounded by sparse northern forests. Pollen data ( Fig. 3a ) indicate that following late-glacial tundra vegetation, Betula expanded massively during the early Holocene. Larix appeared about 11,000 calibrated years before present (cal yr BP=1,950) and its maximum extent was between 9,500 and 5,000 cal yr BP. The slight decrease of the Larix cover was paralleled by an expansion of wet understory vegetation as indicated by an increasing Ericaceae and Sphagnum . Variation partitioning using RDA reveals that of the 68.9% explained variation in the diatom data ( Table 2 ), vegetation (scores of principal component analysis (PCA) axes 1 and 2 based on fossil pollen data) uniquely explains a higher amount of variation than insolation (January and July for 69°N), fluvial activity (indicated by sand content), or lake depth (assessed by Fe/Mn ratio). However, most variation is explained by a combination of several environmental variables, indicating a strong coupling of the various components in the system. Reconstructed values of HCO 3 − (based on a newly developed regional diatom–HCO 3 − transfer function, see Methods) are about 100 mg l −1 during the early Holocene but decrease markedly later with a particularly strong decrease ~5,500 cal yr BP to the present values of about 15 mg l −1 . The phase of Larix and Betula maximum cover is characterized by the highest lake alkalinity, which, according to our conceptual model ( Fig. 2 ), originates from higher evapotranspiration rates and enhanced ion import to the lake from surrounding soils and reduced run-off. 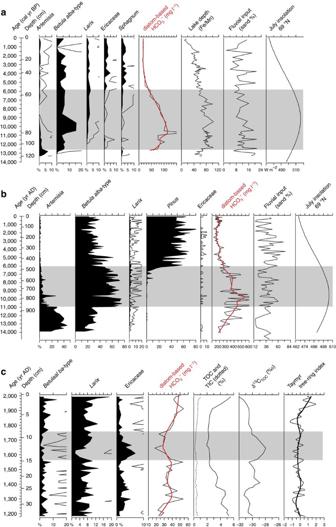Figure 3: Results of sediment investigations from three sites in northern Siberia. (a) Sysy Kyuele, lower Lena river lowlands covered by open northernLarixforests. (b) Ulakhan Chabyda, central Yakutian lowlands in the typicalLarixtaiga zone. (c) Lake SA-34, upper Popigai River on the border between Yakutia and Krasnoyarski Krai, surrounded by northernLarixforests. In the interpretation of our pollen data, we assume thatArtemisiaindicates openness of vegetation,Betula alba-type andLarixindicate forest extent and composition, and Ericaceae andSphagnumindicate the extent of wetland vegetation either in the form of mire patches or in the forest understory. Changes in lake depth and fluvial activity are inferred from the variation in Fe/Mn and sand%. Alkalinity reconstructions are presented in mg HCO3−l−1. It is based on the application of a modern transfer function (model validation by jackknifing yields a root-mean square error of prediction (RMSEP) of 0.3log+1 mg l−1) to fossil diatom assemblages. Major trends are summarized by a LOESS (locally estimated scatterplot smoothing smoother) (span: 0.25). For Lake SA-34, the reconstructed alkalinity changes were validated by changes in the inorganic carbon supply as indicated byδ13C of organic carbon. July insolation (Fig. 2a,b)44or Taymyr tree-ring width chronology (Fig. 2c)19are plotted as independent records of summer temperature changes. Chronologies developed on the basis of radiocarbon dates justify the interpretation of millennial-scale changes at Sysy Kyuele and Ulakhan Chabyda. For Lake SA-34, an age-depth model based on210Pb/137Cs and radiocarbon dates provides a reliable basis to interpret centennial-scale changes. Highlighted in gray are phases of specific interest discussed in the text. Figure 3: Results of sediment investigations from three sites in northern Siberia. ( a ) Sysy Kyuele, lower Lena river lowlands covered by open northern Larix forests. ( b ) Ulakhan Chabyda, central Yakutian lowlands in the typical Larix taiga zone. ( c ) Lake SA-34, upper Popigai River on the border between Yakutia and Krasnoyarski Krai, surrounded by northern Larix forests. In the interpretation of our pollen data, we assume that Artemisia indicates openness of vegetation, Betula alba- type and Larix indicate forest extent and composition, and Ericaceae and Sphagnum indicate the extent of wetland vegetation either in the form of mire patches or in the forest understory. Changes in lake depth and fluvial activity are inferred from the variation in Fe/Mn and sand%. Alkalinity reconstructions are presented in mg HCO 3 − l −1 . It is based on the application of a modern transfer function (model validation by jackknifing yields a root-mean square error of prediction (RMSEP) of 0.3log+1 mg l −1 ) to fossil diatom assemblages. Major trends are summarized by a LOESS (locally estimated scatterplot smoothing smoother) (span: 0.25). For Lake SA-34, the reconstructed alkalinity changes were validated by changes in the inorganic carbon supply as indicated by δ 13 C of organic carbon. July insolation ( Fig. 2a,b ) [44] or Taymyr tree-ring width chronology ( Fig. 2c ) [19] are plotted as independent records of summer temperature changes. Chronologies developed on the basis of radiocarbon dates justify the interpretation of millennial-scale changes at Sysy Kyuele and Ulakhan Chabyda. For Lake SA-34, an age-depth model based on 210 Pb/ 137 Cs and radiocarbon dates provides a reliable basis to interpret centennial-scale changes. Highlighted in gray are phases of specific interest discussed in the text. Full size image Lake Ulakhan Chabyda core and transitions among forest types Evapotranspiration differs markedly among different forest types. Comparisons among Larix - and Pinus -dominated stands show that in accordance with the higher leaf-area index of Larix compared with that of the Pinus , the sapflow rate of single Larix trees is higher [16] . We assume that differences in mean ion content of lakes from different forest types (from low to high— Pinus , Larix and Betula, Supplementary Fig. S1 ), at least partly, originate from differences in evapotranspiration rates, as confirmed by differences in soil carbonate and soluble salt content among sites [11] . Our sediment analyses at Ulakhan Chabyda in the central Yakutian lowlands support this hypothesis. In its surroundings, Larix was probably dominant and Betula obtained high cover from around 9,500–5,500 cal yr BP ( Fig. 3b ). Invasion of Pinus started from about 7,000 cal yr BP, and from about 6,000 cal yr the lake’s surroundings were covered by Pinus – Larix forests similar to the present day. Modern analogue matching for fossil Ulakhan Chabyda samples shows that good analogues are available from the central Yakutian Larix forest sites for the period since ~6,000 cal yr BP when modern conditions became established around Ulakhan Chabyda ( Supplementary Fig. S4 ). However, the closest modern analogues for the earlier period occur in the present-day central Mongolian Larix–Betula forest zone [17] . Diatom-based reconstructions show that HCO 3 − concentrations temporarily reached 900 mg l −1 during the early Holocene, with a marked decrease from 7,100 to 4,500 cal yr BP to ~150 mg l −1 today. Accordingly, we assume that the much higher abundance of Betula during the early-to-mid Holocene (also seen at Sysy Kyuele), and related higher evapotranspiration, contributed to the higher lake ion content. At Ulakhan Chabyda, this trend was enhanced by the mid-Holocene Pinus invasion on sandy soils characterized by a low permafrost table that was probably formerly covered by Betula . Time scales of change To test whether the millennial-scale processes mirrored by the records described above apply to centennial to decadal time scales, which would enhance the implications of our conceptual model for future ecosystem changes, we investigated a short core from a small lake in the Popigai catchment, in the area between northwestern Yakutia and Krasnoyarski Krai, presently surrounded by the northern Larix forests ( Fig. 1 ). A comparison of the pollen and diatom results reveals a significant correlation between changes in vegetation and phytoplankton ( Fig. 3c ). Expansion of Ericaceae in the forest understory of the northern Larix forests during the seventeenth century, indicating moister soil conditions, is paralleled by decreasing lake alkalinity as indicated by very low diatom-based HCO 3 − concentrations, low total inorganic carbon (TIC) values and high δ 13 C of total organic carbon (TOC), the latter originating from a limitation in carbon supply in the water column [18] . When compared with a regional tree-ring chronology [19] , this minimum coincides with below-average ring widths, potentially originating from cold summers on the onset of the Little Ice Age. The twentieth century, in contrast, was characterized by high summer temperatures and high Larix percentages, and was compared with the seventeenth century average, a doubling of lake HCO 3 − concentrations. Our results have several implications that are not yet considered with respect to the status of larch taiga ecosystems (and of northern forests in general) in response to future global warming. According to our modern analyses, thaw lakes represent a major reservoir of inorganic carbon. GIS analyses ( Supplementary Methods ) reveal that about 40% of the Yakutia (~size of continental Europe) are lowlands ( Fig. 1 ) typically covered by ice-rich permafrost sediments [15] . According to the global lake database [20] for lakes >1 km 2 and that predicted from a power-law fitted to lakes between 1 and 0.1 km 2 , the tundra, northern forests and typical taiga lowlands cover ~13%, 10% and 5%, respectively, of the catchments of lakes with an area >0.1 km 2 . If we assume these lakes are, respectively, 3.1, 3.0 and 2.3 m deep (median depths in our database), the present-day dissolved inorganic carbon content approximately sums to 0.004 Pg C when we apply the observed median HCO 3 − concentrations of 16, 98 and 278 mg l −1 for the tundra, northern forests and taiga lakes. If we assume that the lake area and depth and the lake-to-latitude distribution during the early or mid-Holocene were similar to today (which represents a rather conservative estimate, as there is evidence that most lakes were deeper and also that thermokarst activity was higher [21] ), and if we assume that the inorganic carbon load in these lakes has increased fivefold (as indicated by changes in our two investigated lakes and in another lake from the Lena Delta [22] ), an extra ~0.02 Pg C is stored in the inorganic carbon reservoir of Yakutian permafrost lakes. In contrast to the rather fixed organic carbon reservoir in permafrost, this fraction is rapidly exchangeable in a climate-driven vegetation change. If terrestrial vegetation is a more direct driver of aquatic ecosystems than thermal regime, this has important implications for aquatic communities under rapid warming. In contrast to an expected immediate response to warming [23] , the time-lagged response of vegetation to climate will result in a climate–aquatic ecosystem disequilibrium. In particular, high-latitude forest establishment is assumed to lag significantly behind a temperature rise [24] , which might result in the formation of new ‘interim’ or novel terrestrial ecosystems dominated by shrubby vegetation [25] . The implication for aquatic environments in the futures is, however, unknown. Even now, freshwater availability is a matter of concern in central Yakutia [26] , a problem that will be of particular relevance to areas farther north under future warming and related vegetation transition [9] . In general, our conceptual model ( Fig. 2 ) contradicts earlier assumptions that with forest expansion during the Holocene, soil acidity and, thus, humic-acid export to lakes increases [27] . Our results support inferences from other studies [28] that processes other than tree immigration into catchments, such as mire expansion or fire, were the drivers of observed lake acidification. The question arises whether the functional coupling between lake ion content and forest density, which we propose in Yakutia is a circum-arctic phenomenon. Treeline transect studies of permafrost-influenced lakes in Alaska and the Northwestern Territories of Canada [29] , [30] , [31] likewise show that ion content and/or alkalinity increase from tundra to forest sites. However, the observed gradients are much smaller than those in Yakutia. These patterns have not been interpreted in terms of a causal relationship with vegetation evapotranspiration rates. They have been tentatively interpreted as a result of higher catchment weathering and organic matter decomposition rates, and increased precipitation [29] , [30] , [31] . Because of the limited comparability of the physical and ecological conditions in eastern Siberia and northwestern North America (for example, Picea and Abies instead of Larix as dominant trees and no continuous permafrost in forested areas in the North American Arctic), it remains speculative whether our proposed functional entity between forests and thaw-lake ion contents is applicable to other arctic sites. In conclusion, we propose that interactions between permafrost, larch forest and thaw lakes represent a missing link in understanding the mineral and inorganic carbon cycling in the lowlands of Siberian taiga forests and that thaw lakes represent a major and, on millennial to decadal scales, highly variable carbon reservoir. Modern sediment material We collected water and surface sediments from 201 lakes scattered throughout Yakutia ( Fig. 1 ) along the whole latitudinal vegetation gradient [32] : 61 lakes are located in the arctic tundra (21 in the forest–tundra zone), 23 lakes in the northern Larix forest and 103 lakes in a typical taiga zone (15 in Pinus – Larix forests, 13 in Betula – Larix forests and 75 in Larix forests). In addition, 14 lakes from mountain forests were sampled. Samples from lakes surrounded by the azonal river valley vegetation were not included. Lakes were sampled in summer 2000–2009. Surface sediments were obtained from the deepest part of each lake using a sediment grab or a gravity corer. The deepest part of each lake was located using a portable echo sounder. Environmental parameters of modern sampling sites Limnological parameters, such as pH, electrical conductivity, lake area, maximum lake depth and Secchi depth, were measured in the field. Water samples were collected from 0.5 m below the surface of each lake, immediately before the retrieval of the sediment samples. The water samples were kept cool during field work and were analysed immediately on return. For ion analysis, water was passed through a cellulose-acetate filter. Samples for cation analysis were then acidified with HNO 3 , whereas samples for anion analysis and residue samples were stored cool. The cation content of the water was analysed by inductively coupled plasma optical emission spectrometry (Perkin-Elmer Optima 3000 XL), whereas the anion content was determined by ion chromatography (Dionex DX-320). Alkalinity was measured using a Metrohm Basic Titrino 794 and the results were evaluated against those obtained in the field using the Alkalinity AL7 titration test kit of Macherey-Nagel. Ion balance was calculated for each sample to validate the analytical methods, resulting in deviations of less than ±5% for most samples. We are aware that PO 4 3− concentrations might have altered significantly during the period between sampling and analysis, but we include these data in the numerical analysis, as they provide general information on important nutrient concentrations. We used the 1 km 2 -MODIS data sets from the ESA DUE Permafrost project [33] to calculate the leaf-area index for our studied sites using the 10-year (2000–2009) mean (excluding all zero values) of the main vegetation period (weekly, 07/10–8/10) for a circular buffer zone of 30 km diameter. Finally, the square-root of the median of all cells was used for further analyses. All this work was done with ArcGIS 10. Mean July temperatures were extracted from a gridded global data set [34] . Diatom analyses Diatom analyses were conducted on about 0.5 g of sediment. The calcareous and organic components were removed by heating with HCl (10%) and H 2 O 2 (30%). Cleaned diatom samples were mounted on microscope slides with Naphrax. About 500 diatom valves per slide were counted along randomly selected transects. The samples were analysed using a Zeiss microscope equipped with a differential interference contrast at a magnification of × 1,000. Water and diatom data of the 103 lakes from Central Yakutia are published by Pestryakova et al. [35] Sediment core material A core of 121 cm length was collected from Sysy Kyuele (69.404°N; 123.828°E; 81 m a.s.l.) in summer 2009. The sediment consists of a sequence from greyish silt to brown organic-rich gyttja. The age-depth model, sedimentological data and the diatom data are published by Biskaborn et al. [36] The 1,060-cm long sediment core from Ulakhan Chabyda (61.98°N; 129.39°E, 218 m a.s.l.) consists of silty lake mud. Pollen and diatom data are published by Andreev et al. [37] and Pestryakova et al. [35] , respectively. A 34-cm length sediment core was collected from lake SA-34 (71.501°N and 110.900°E, 85 m a.s.l. ), using a gravity corer. Granulometric and organic carbon analyses (not shown) indicate that sediments consist of silty lake mud without major changes. 210 Pb measurements indicate that the upper 5.7 cm accumulated after 1860 AD and within error ranges the 1963-AD- 137 Cs-maximum verifies this chronology ( Supplementary Figs S5, S6, S7 , Supplementary Tables S2, S3, S4 and Supplementary Note 1 ). The chronology of the lower part of the core is based on the age-depth model using radiocarbon dates. We used the BACON software [38] on twelve 14 C dates to construct a robust age-depth model (for details, see Supplementary Note 1 ). The reliability of the inferred ages from the lower part is supported by an almost similar age-depth model generated from the extrapolation of the mean sedimentation rate inferred from 210 Pb dating of the upper part of the core. Statistical analyses All lake-water chemical and sedimentary variables were transformed using log(x+1) (with the exception of pH) and were standardized. Diatom data were expressed as relative abundances. Species were retained in numerical analysis if they occur in at least six modern lake samples with an abundance of >0.5%, or if they occur in at least one lake with an abundance of >20%. The following analyses were performed: principal component analysis (PCA), which was run on the ion composition data to investigate relationships among the different ions. On the basis of the arrow length and position in the ordination biplot, a set of three variables (HCO 3 − , Cl − and Si) was selected for further analyses to avoid effects from collinearity of the various chemical parameters (a full list of all parameters and the biplot is shown in the Supplementary Fig. S1 ). RDA, which is a powerful constrained ordination method to detect the explanatory power of a single or a group of predictor variables for a multivariate data set of response variables that have predominantly linear relationships with the predictor variables, was executed. Three sets of RDA were run to investigate the relationships as follows: first, between the modern lake ion composition and environmental variables (leaf-area index, mean July temperature, and lake depth and area); second, between modern diatom data and site-specific environmental characteristics (selected chemical variables and lake depth and area); and third, between fossil diatoms from Sysy Kyuele and independent proxies for vegetation (samples scores on the first two PCA axes of pollen data that were found to be significant when testing against a broken-stick model), lake depth (Fe/Mn ratio) and fluvial activity (sand %). In a first step, all environmental variables were included to infer the total amount of variation that can be explained by the environmental ‘predictor’ variable set. In a second step, we performed variation partitioning to explore the amount of variation in the compositional data that is uniquely explained by each single environmental variable (by including the other variables as covariables). For the modern diatom data set, additional RDA runs, including each chemical parameter separately, were performed to identify the most relevant environmental variable that could be used for quantitative environmental inferences. Scaling focuses on intervariable correlations in all ordinations. Monte Carlo permutation tests to indicate significance at the P <0.05 level were performed under the full model, with 999 permutations. PCA and RDAs were performed using CANOCO version 4.5 (ref. 39 ), and the broken-stick model [40] was carried out using the biodiversity R package. Quantitative transfer functions for inferring alkalinity (that is, the concentration of HCO 3 − ) from fossil diatom assemblages were developed using weighted-averaging partial least-squares regression. Surface samples from sites that were later used for reconstructions were excluded from the calibration set. In addition to our data from Yakutia, a diatom data set of 26 Mongolian lakes [17] was included to improve potentially the reliability of the reconstructions of late glacial–early Holocene conditions at Ulakhan Chabyda where a high abundance of Cyclotella radiosa was recorded, which has no modern analogues in the modern Yakutian data set. Weighted-averaging partial least-squares regressions were implemented with C2 software version 1.3 (ref. 41 ). A one-component model was selected, as it has a high r 2 (0.77) and a low root-mean square error of prediction (0.30 log(x+1) mg l −1 ) ( Supplementary Fig. S8 ), and as the performance of a two-component model was not a statistically significant improvement over the one-component model (randomization t -test P >0.13). The final transfer functions were applied to fossil diatom spectra from Sysy Kyuele and Ulakhan Chabyda. The reconstructed values of the core tops of 1.2 log(x+1) mg l −1 for Sysy Kyuele and 2.3 log(x+1) mg l −1 for Ulakhan Chabyda are in reasonably good agreement with the present-day measured HCO 3 − concentrations of 1.1 and 2.4 log(x+1) mg l −1 , respectively. As, according to the pollen data, vegetation variability during the last millennium at SA-34 did not cover the whole environmental range of present-day Yakutia, a submodel was used for the reconstruction of lake SA-34’s alkalinity, where only sites from northern forests, tundra and mountainous forests (99 lakes) were included, which yielded a slightly lower root-mean square error of prediction of 0.26 log(x+1) mg l −1 but markedly improved model predictions at the low mineralized sites. To assess the reliability of the reconstructed values, analogue matching was performed with squared-chord distance (SCD) as the dissimilarity measure [42] , [43] . Plots of minimum distance versus age indicate ( Supplementary Fig. S4 ) that almost all samples have very good or good analogues in the modern data set (that is, meet the 1% percentile located at 0.56 SCD or the 2.5% percentile at 0.69 SCD, respectively). A few samples from Ulakhan Chabyda around 7,000 cal yr BP are characterized by a high Navicula diluviana abundance, which is absent from the modern Yakutian diatom flora and thus have only poor analogues in the modern diatom data set. Furthermore, high Ellerbeckia arenaria abundances observed in some of the levels in the lake SA-34 record are rarely found in modern assemblages. However, these samples do not impact the general inference of the alkalinity reconstructions presented here. How to cite this article: Herzschuh, U. et al. Siberian larch forests and the ion content of thaw lakes form a geochemically functional entity. Nat. Commun. 4:2408 doi: 10.1038/ncomms3408 (2013).